Reversible nano-structuring of SrCrO3-δthrough oxidation and reduction at low temperature Oxygen vacancies are often present in complex oxides as point defects, and their effect on the electronic properties is typically uniform and isotropic. Exploiting oxygen deficiency in order to generate controllably novel structures and functional properties remains a challenging goal. Here we show that epitaxial strontium chromite films can be transformed, reversibly and at low temperature, from rhombohedral, semiconducting SrCrO 2.8 to cubic, metallic perovskite SrCrO 3- δ . Oxygen vacancies in SrCrO 2.8 aggregate and give rise to ordered arrays of {111}-oriented SrO 2 planes interleaved between layers of tetrahedrally coordinated Cr 4+ and separated by ~1 nm. First-principle calculations provide insight into the origin of the stability of such nanostructures and, consistent with the experimental data, predict that the barrier for O 2− diffusion along these quasi-two-dimensional nanostructures is significantly lower than that in cubic SrCrO 3- δ . This property is of considerable relevance to solid oxide fuel cells in which fast O 2− diffusion reduces the required operating temperature. The fascinating properties of oxides, specifically perovskites, are often discussed in terms of partially occupied transition metal (TM) d orbitals and corresponding local atomic structures [1] . Oxygen vacancy ( V O ) formation simultaneously induces changes in coordination and in the formal charge of the nearest TM cations. However, V O can also affect the electronic properties and structural environment of TM cations that are further away. If V O are present in sufficiently high concentrations, they can in principle aggregate and form new ordered structures, such as charge and spin density waves, with or without corresponding structural rearrangements. Significantly, such ordered structures can have properties not observed in the host lattice, and can be regarded as novel, mesoscale crystals [2] , [3] . Here we report that accumulation of V O in the cubic perovskite SrCrO 3 (P-SCO) results in the formation of ordered, nanostructured, rhombohedral SrCrO 2.8 (R-SCO) with quite different electronic and optical properties. We also demonstrate that R-SCO can be reversibly oxidized to P-SCO under mild and easily controlled experimental conditions, and that the R-SCO structure gives rise to much more facile oxygen ion (O 2− ) conductivity than that in P-SCO. This property is exceedingly important for solid oxide fuel cell technology, where oxygen reduction reaction kinetics and oxide ion conductivity in the cathode currently require high temperatures (~800 °C) that significantly lower overall energy efficiency [4] , [5] , [6] . More generally, our results show that isolated V O defects can aggregate into anisotropic, quasi-two-dimensional (2D) structures that are defect free, and might allow the spatial separation of electronic and vibrational degrees of freedom, which would be useful in, for example, thermoelectric applications. Structural modifications in the reduced phase Under the same conditions that lead to fully oxidized LaCrO 3 (ref. 7 ), the deposition of epitaxial P-SCO on (001)-oriented perovskites, such as LaAlO 3 (LAO) and (LaAlO 3 ) 0.3 –(SrAl 0.5 Ta 0.5 O 3 ) 0.7 (LSAT), by means of molecular beam epitaxy, results in R-SCO. Conversion of R-SCO to P-SCO occurs during mild heating in air. Evidence for this phase transition is given by X-ray diffraction (XRD), as seen in Fig. 1a and Supplementary Fig. 1a . All as-grown films exhibit a single Bragg peak at 2 θ ≈46° near the substrate (002) reflection, revealing epitaxy. These Bragg angles increase substantially upon annealing in air, revealing a sizeable drop in c lattice parameter. The changes in lattice constants (based on reciprocal space maps—see Supplementary Figs 1 and 2 ) are summarized in Fig. 1b . The in-plane lattice parameters for the as-grown films (3.82 Å on LAO and 3.86 Å on LSAT) are nearly the same as those of their respective substrates, whereas the out-of-plane lattice constant ( c ) is ~3.92 Å for both films on both substrates. The larger value of c in the as-grown films compared with that of bulk SrCrO 3 (3.819 Å) implicates the presence of V O through a phenomenon called chemical expansivity [8] , [9] . The drop in c upon air annealing is consistent with oxidation of R-SCO to P-SCO. 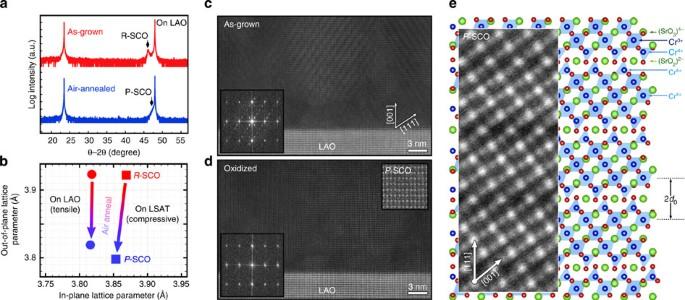Figure 1: Topotactic phase transition of strontium chromite from rhombohedral SrCrO2.8(R-SCO) to cubic perovskite SrCrO3-δ. (a) XRDθ–2θscans of the as-grown R-SCO film on LAO(001) (red curve) that transforms into cubic perovskite SrCrO3-δafter annealing in air at 250 °C for 2 h (blue curve). (b) Evolution of the in-plane and out-of-plane lattice constants for the epitaxial films obtained from reciprocal space maps around the (103) Bragg reflection of the substrates; circles and squares represent films grown on LAO and LSAT, respectively. (c) Cross-sectional high-angle annular dark field (HAADF)-scanning transmission electron microscopy (STEM) image as viewed along [110] for as-grown R-SCO film on LAO(001), showing (111)-oriented planes of ordered oxygen vacancy planes every five unit cells along [111], both in the image (dark stripes) and by the superlattice peaks in the FT (inset). (d) After annealing in air at 250 °C, the ordered vacancies are substantially eliminated, resulting in P-SCO (upper right inset) and the corresponding disappearance of the superlattice reflections (lower left inset). (e) HAADF-STEM image (averaged over many short exposures) revealing an ordered oxygen-deficient structure that is well matched to a 15Runit cell with periodic (111)-planes of Cr4+tetrahedra, overlaid on a calculated structural model structure (see text for details). Figure 1: Topotactic phase transition of strontium chromite from rhombohedral SrCrO 2.8 (R-SCO) to cubic perovskite SrCrO 3- δ . ( a ) XRD θ– 2 θ scans of the as-grown R-SCO film on LAO(001) (red curve) that transforms into cubic perovskite SrCrO 3- δ after annealing in air at 250 °C for 2 h (blue curve). ( b ) Evolution of the in-plane and out-of-plane lattice constants for the epitaxial films obtained from reciprocal space maps around the (103) Bragg reflection of the substrates; circles and squares represent films grown on LAO and LSAT, respectively. ( c ) Cross-sectional high-angle annular dark field (HAADF)-scanning transmission electron microscopy (STEM) image as viewed along [110] for as-grown R-SCO film on LAO(001), showing (111)-oriented planes of ordered oxygen vacancy planes every five unit cells along [111], both in the image (dark stripes) and by the superlattice peaks in the FT (inset). ( d ) After annealing in air at 250 °C, the ordered vacancies are substantially eliminated, resulting in P-SCO (upper right inset) and the corresponding disappearance of the superlattice reflections (lower left inset). ( e ) HAADF-STEM image (averaged over many short exposures) revealing an ordered oxygen-deficient structure that is well matched to a 15 R unit cell with periodic (111)-planes of Cr 4+ tetrahedra, overlaid on a calculated structural model structure (see text for details). Full size image The R → P conversion is clearly seen by cross-sectional, high-angle annular dark field scanning transmission electron microscopy (TEM). Domains with {111}-ordered planar superlattice structures are observed, seen as dark stripes repeating every five unit cells in Fig. 1c . The ordered {111}-plane domains generate a set of superlattice spots in the Fourier transforms (FT; inset in Fig. 1c ). Figure 1e shows a more magnified lattice image, along with the structural model discussed below. The positions of visible Cr and Sr atomic columns are consistent with {111}-oriented SrO 2 layers separated by four SrO 3 layers. This ordered structure (a 15 R polymorph) is the same as that of R-SCO that forms upon reduction of P-SCO powder [10] . As in ref. 10 , we find that Cr adjacent to the SrO 2 planes is tetrahedral Cr 4+ , whereas the other three Cr layers located between SrO 2 planes contain Cr with an average charge of +3.33; these ions retain the octahedral coordination found in P-SCO. The distribution of Cr charge states throughout the structure was imaged by electron energy loss spectroscopy (EELS). EELS maps tracking the near-edge structure of the Cr L-edge, as shown in Supplementary Fig. 3 , is consistent with Cr 4+ being detected within the SrO 2 -containing stripes and Cr 3+ being found between these stripes, based on a reported 1 eV chemical shift between Cr 3+ in LaCrO 3 and Cr 4+ in CrO 2 (ref. 11 ). Based on this experimental data and ab initio calculations, it is natural to consider the crystal structure of R-SCO in terms of 〈111〉-oriented lamella consisting of , where and have charges of −1 and +2 with respect to the lattice. The packing of these lamella can be understood in terms of the electrostatic interactions between atomic planes. Ab initio calculations reveal that two such lamellae do not interact if separated by five or more Cr planes ( Supplementary Fig. 4 ). The repulsion energy of two lamellae separated by only four Cr planes is ~0.45 eV per (1 × 1) lateral 15 R cell, and it rapidly rises as the distance between the [SrO 2 ] 2– planes decreases and lamellae begin to overlap. This result is consistent with the experimentally observed structure, and suggests that under reducing conditions the ordered oxygen-deficient layers pack as closely as possible without incurring a repulsive energy penalty, and implies that these 2D structures are mobile and can move along the 〈111〉 direction, either in aggregate or as isolated vacancies. Provided the spacing between lamellae ( d 1 ) exceeds the spacing between a central SrO 2 layer and it nearest octahedral Cr 3+ layer ( d o ), there is no repulsion between the two lamellae. Evidence for reversible reduction/oxidation processes The majority of the oxygen-deficient planes are removed by annealing in air for 2 h at only 250 °C as, accordingly, R-SCO is transformed into P-SCO, as clearly seen in the scanning TEM image and FT (inset) in Fig. 1d . This phase transformation involves two processes: (1) insertion of oxygen atoms into SrO 2 layers to form SrO 3 , and (2) electron transfer from octahedrally coordinated Cr 3+ ions located between the SrO 2 layers so as to convert the inserted oxygen atoms into O 2– ions. As oxidation proceeds, XRD reveals a contraction in the out-of-plane lattice constant by ~2% ( Fig. 1a,b ). The (103) Bragg reflection for the air-annealed sample indicates that the lattice constant is close to that of the bulk P-SCO ( Supplementary Fig.2 ). Therefore, we refer to the air-annealed sample as P-SrCrO 3- δ . It is difficult to determine the exact value of δ because O vacancies distribute randomly and their concentration is very low; our ab initio calculations indicate that δ should be ≤0.10 in order to form the P-SCO phase. This oxidation process can be dynamically observed in situ with high spatial resolution using environmental TEM (ETEM). The vacancy planes are eliminated by annealing at 250 °C in 1.5 mbar oxygen gas within ~30 min. To ensure that the apparent oxidation is not a result of beam damage, the sample was imaged at the same temperature and pressure in Ar for ~45 min before introducing oxygen with no apparent changes observed during this time. In oxygen at 250 °C, the oxygen-deficient domains typically vanish more quickly than could be captured in our apparatus (<10 frames per second under imaging conditions). In order to slow the process, experiments were also performed by introducing a partial pressure of 0.05 mbar oxygen at 400 °C. The individual ordered oxygen-deficient SrO 2 planes still oxidize very quickly, but single domains sometimes heal in steps ( Supplementary Movie 1 ). Incorporation of oxygen may go unnoticed until a sudden R-to-P phase transition occurs, as the relevant TEM contrast is more sensitive to the structural discontinuity than to the individual oxygen ions. The grouping of rapidly oxidized SrO 2 planes seems to correlate with the location of {111}-oriented structural defects formed at, for example, grain boundaries between mutually orthogonal {111}-ordered domains ( Supplementary Fig. 5 ). This result suggests that the oxidation rate is limited by defect formation. As oxygen is incorporated into the SrO 2 layers, the local structure changes and the superlattice diffraction spots in the FT disappear. In addition, the out-of-plane lattice parameter decreases by 1.7%, and the in-plane parameter decreases by 0.8%. This result is consistent with XRD data and the results of our Perdew-Burke-Ernzerhoff (PBE) calculations for unconstrained SrCrO 3- δ , which suggest that the R-to-P structural transition is accompanied by an out-of-plane lattice parameter decrease of 3.2–3.6%, depending on the residual V O concentration, while the in-plane lattice parameter decreases by 1.1–1.5%. Spectroscopy and the semiconductor-to-metal transition Cr 2 p core-level and valence band (VB) X-ray photoemission spectra, along with conductivity and optical absorption, reveal the expected changes in Cr valence and the electronic structure of the SCO lattice as a whole as the phase transition takes place. 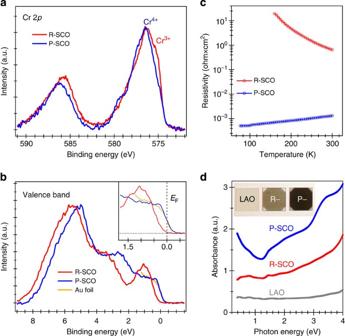Figure 2: Significant differences in electronic and optical properties for the R and P phases. (a) Cr 2pcore-level spectra for as-grown (R-SCO) and air-annealed (P-SCO) films on LAO(001), showing that the Cr3+contributions to both spin-orbit components are significantly reduced by air annealing. (b) X-ray-excited VB photoemission spectra for the as-grown and air-annealed films. Inset shows the spectra near the Fermi level (EF), along with the spectrum from an Au foil in direct contact with the films for energy calibration purposes. There is little intensity atEFfor as-grown films, whereas substantial intensity appears atEFfor air-annealed films, indicating a semiconductor-to-metal transition. (c) Temperature-dependent resistivityρ(T) curves for as-grown and air-annealed films, revealing semiconducting behaviour for R-SCO and metallic behaviour for P-SCO. (d) Optical absorption spectra for the as-grown and air-annealed films, as well as an LAO substrate. Figure 2a shows that for R-SCO, there is, in addition to a main peak at ~576.5 eV associated with Cr 4+ , a strong shoulder at ~575.2 eV attributed to Cr 3+ (ref. 7 ). After air annealing, the intensity of this shoulder is significantly reduced as the P-SCO phase forms, corresponding to oxidation of Cr 3+ to Cr 4+ as the phase transition occurs. This change in Cr valence is accompanied by distinct changes in the electronic and optical properties of the film. Temperature-dependent resistivity ρ(T) data, shown in Fig. 2c and Supplementary Fig. 1c , indicate that R-SCO is semiconducting (d ρ/ d T <0), whereas P-SCO is metallic (d ρ/ d T >0). In addition, the resistivity of P-SCO (2 × 10 −3 Ω cm) is almost three orders of magnitude smaller than that of R-SCO (6 × 10 −1 Ω cm). This marked change in resistivity is accompanied by a colour change from transparent grey to opaque dark ( Fig. 2d , inset). The optical absorption spectra for R-SCO films show no discernible absorption below hν =2.0 eV, consistent with its semiconductor behaviour. In contrast, P-SCO exhibits a strong absorption onset for hν less than ~1.0 eV, consistent with light scattering by carriers in the metallic phase. Figure 2: Significant differences in electronic and optical properties for the R and P phases. ( a ) Cr 2 p core-level spectra for as-grown (R-SCO) and air-annealed (P-SCO) films on LAO(001), showing that the Cr 3+ contributions to both spin-orbit components are significantly reduced by air annealing. ( b ) X-ray-excited VB photoemission spectra for the as-grown and air-annealed films. Inset shows the spectra near the Fermi level ( E F ), along with the spectrum from an Au foil in direct contact with the films for energy calibration purposes. There is little intensity at E F for as-grown films, whereas substantial intensity appears at E F for air-annealed films, indicating a semiconductor-to-metal transition. ( c ) Temperature-dependent resistivity ρ ( T ) curves for as-grown and air-annealed films, revealing semiconducting behaviour for R-SCO and metallic behaviour for P-SCO. ( d ) Optical absorption spectra for the as-grown and air-annealed films, as well as an LAO substrate. Full size image The VB spectrum for R-SCO ( Fig. 2b ) is primarily of O 2 p character in the region of 2.2–8.5 eV, and exhibits a Cr 3 d -derived feature at ~1.0 eV. There is only very slight spectral intensity detected at the Fermi level ( E F ) ( Fig. 2b , inset), suggesting semiconducting behaviour. In contrast, pronounced intensity at E F is seen for P-SCO, revealing its metallic character. It is noteworthy that the physical properties of SrCrO 3 are controversial. A critically important issue is whether SrCrO 3 is metallic or insulating [12] , [13] , [14] . This controversy most likely exists because of poorly defined structure and/or composition in powder samples. Our experimental results provide definitive evidence that single-crystal stoichiometric SrCrO 3 is metallic. The metallic state of P-SCO is attributed to strong hybridization of the Cr 3 d 2 t 2g configuration with O 2 p states, which results in delocalized holes at the top of the VB. Cr 3 d -O 2 p hybridization and hole delocalization are further supported by the presence of an intense pre-edge peak in the O K-edge EELS ( Supplementary Fig. 6 ). This assignment is consistent with those for SrCoO 3 (ref. 15 ) and SrFeO 3 (ref. 16 ), as well as CrO 2 (ref. 17 ). Remarkably, the P-SCO to R-SCO phase transition is fully reversible at moderately low temperature. P-SCO can be transformed back into R-SCO by annealing in vacuum at 500 °C for 1 h, as confirmed by XRD and ρ ( T ) data ( Supplementary Fig. 7 ). Likewise, R-SCO can be re-oxidized to P-SCO by annealing in air at 250 °C. Using photoemission intensity at E F to monitor metallicity, the redox process was followed during in vacuo and air annealing. The results are shown in Fig. 3a . The count rate at E F starts to decrease as a result of vacuum annealing at 300 °C, and goes to zero at 500 °C after 1 h, revealing a metal-to-insulator transition. The Cr 2 p core-level and VB spectra for the 500 °C vacuum-annealed sample are similar to those for the as-grown R-SCO ( Supplementary Fig. 7b,c ). Upon annealing in air at 200 °C or below, there is no significant change in the intensity at E F ( Fig. 3a , blue). However, the R-to-P phase transition starts at 250 °C. These results illustrate that the V O concentration can be used to tune the conductivity of complex oxides in a way analogous to the role of dopants in conventional semiconductors with two important distinctions. First, in the case of V O in oxides, the doping process is reversible, revealing a way to dynamically control functionality not possible in conventional semiconductors [18] . Second, isolated anion vacancies are typically n -type dopants that result in higher electron conductivity. However, in the case of SCO, V O result in a lower conductivity because the electrons associated with V O populate a partially occupied t 2g sub-band of Cr, and thus decrease the number of charge carriers and increase optical transparency. 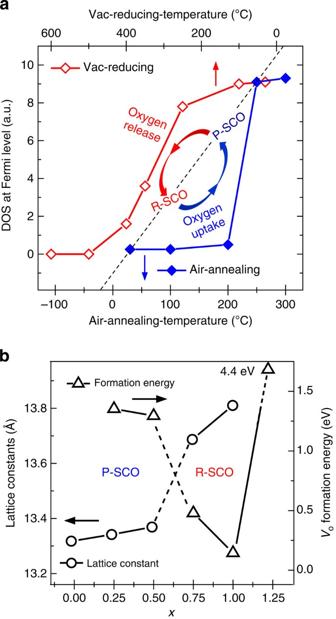Figure 3: Cyclical oxidation and reduction of SrCrO3-δvia the R↔P phase transition. (a) Photoemission intensity at the Fermi level as a function of annealing temperature in air (blue curve) and in vacuum (red curve), indicating that the R-SCO to P-SCO transition (oxidation) occurs at 200–250 °C and the P-SCO to R-SCO transition (reduction) occurs at 500 °C. (b) Calculated O vacancy formation energies and lattice parameters as function of oxygen vacancy concentration in an isolated {111}-oriented SrO3–xplane. Figure 3: Cyclical oxidation and reduction of SrCrO 3- δ via the R↔P phase transition. ( a ) Photoemission intensity at the Fermi level as a function of annealing temperature in air (blue curve) and in vacuum (red curve), indicating that the R-SCO to P-SCO transition (oxidation) occurs at 200–250 °C and the P-SCO to R-SCO transition (reduction) occurs at 500 °C. ( b ) Calculated O vacancy formation energies and lattice parameters as function of oxygen vacancy concentration in an isolated {111}-oriented SrO 3– x plane. Full size image The propensity of P-SCO to reduce to R -SCO has thermodynamic origins. High oxygen pressure is needed to synthesize bulk SrCrO 3 (ref. 13 ) and rutile CrO 2 (ref. 19 ). The octahedral environment of Cr 4+ in cubic perovskite is metastable and would relax to a lower symmetry configuration. In contrast, both Cr 3+ O 6 octahedra and Cr 4+ O 4 tetrahedra are stable at ambient conditions [20] . To characterize the thermodynamic stability of SCO, we calculated the formation energies of V O in SrCrO 3– δ as a function of δ , shown in Fig. 3b . According to these calculations, forming an isolated V O requires 1.3 eV, a very low value compared with La-based perovskites, for example, LaCrO 3 (3.9 eV), and lower than that found for other Sr B O 3 perovskites with an incomplete B t 2g shell, for example, SrCoO 3 (~1.6 eV; ref. 21 ). When there are ≤2 V O per supercell ( δ ≤0.10), the perovskite structure is preserved even if the vacancies are located in the same {111}-oriented SrO 3 lattice plane; the lattice parameters expand by 0.4% on average with respect to those of stoichiometric SrCrO 3 . The energy required to form the third vacancy ( δ =0.15) depends strongly on its location relative to other V O . In the most stable configuration we considered, the three vacancies occupy sites in the same Sr 4 O 12 plane of the supercell, perpendicular to the 〈111〉 axis in the manner consistent with the results of our TEM observations ( Fig. 1e ) and the corresponding vacancy formation energy is only 0.5 eV. Furthermore, this plane, which becomes Sr 4 O 9 after the P-to-R phase transition is completed, undergoes significant relaxation. In particular, seven out of nine remaining oxide ions displace such that Cr cations in neighbouring planes become tetrahedrally coordinated, the separation between the Cr planes increases from 2.22 Å in stoichiometric SrCrO 3 to 2.88 Å, and the lattice transforms to rhombohedral. Unlike in the case of isolated vacancies, the six electrons associated with the three V O localize on the Cr cations not in the first but in the second-nearest plane to the Sr 4 O 9 plane of the supercell. Thus, the width of this quasi-2D oxygen-deficient structure corresponds to the space occupied by four consecutive 〈111〉-oriented Cr planes. Formation of one more V O in this Sr 4 O 9 plane ( δ =0.20) requires only 0.15 eV, which clearly shows that segregation of isolated oxygen vacancies into quasi-2D structures is thermodynamically favourable. After relaxation of the resulting Sr 4 O 8 plane (SrO 2 plane per 1 × 1 lateral cell), all neighbouring Cr cations are tetrahedrally coordinated and retain their 4+ charge state, whereas the second-nearest Cr cations remain octahedrally coordinated and adopt a charge of 3+. In addition, the in-plane and out-of-plane cell parameters increase by 1.6 and 3.7% with respect to those of SrCrO 3 , and the separation between the Cr planes across the oxygen-deficient plane becomes 3.03 Å. Finally, we note that once the Sr 4 O 8 plane is stabilized, formation of an additional V O in the same plane is very costly; the corresponding formation energy jumps to 4.4 eV, as seen in Fig. 3b . The R-to-P phase transition thus involves two steps. First, oxygen is reduced and incorporated as O 2− at the surface. Second, O 2− ions diffuse into the film to oxidize SrO 2 planes, forming P-SCO. The diffusion of O 2− at such a low temperature (250 °C) is of particular interest because O 2− conduction typically involves a thermally activated hopping mechanism and requires high temperatures (for example, >~700 °C; refs 22 , 23 ). We theoretically investigated the mechanisms of oxygen diffusion in both P- and R- phases. As expected, diffusion in P-SCO occurs via V O -mediated hopping and involves a relatively large ( a 0 /√2) displacement of a single O 2− ( Supplementary Movie 2 ). The calculated migration energy barrier for this process is 0.5 eV, and similar values were calculated for other oxygen-deficient perovskites [23] . In contrast, O 2− diffusion in R-SCO involves small cooperative displacements of several atoms, bond breaking and formation of new bonds. A single-diffusion event can be considered as a sequence of three elementary steps, as depicted in Fig. 4a,b : (i) breaking a bond between an O and a five-coordinate Cr (Cr 5C ); (ii) displacement of three neighbouring oxide ions; and (iii) formation of a new O–Cr 5C bond. This mechanism is similar to the Grotthuss mechanism of proton diffusion in water [24] , and is clearly different from the conventional vacancy-mediated mechanism of O 2− diffusion in fluorite and perovskite oxides. While the energy barrier for this process depends on lattice parameters, the effect is negligible as long as the R-SCO structure persists. In the case of δ =0.2, this barrier is ~0.15 eV, whereas for δ =0.15, with its slightly smaller lattice parameters, this barrier decreases to ~0.12 eV. The possible diffusion pathways resulting from such elementary steps are illustrated in Fig. 4c,d . Here we show the SrO 2 layer and two adjacent Cr planes only. For every interstitial O 2– site (marked with crosses in Fig. 4d ), there are four possible pathways leading to equivalent locations in the same layer ( Fig. 4c ). The choice between these pathways is determined by the instantaneous tilt angles of the Cr–O bonds oriented perpendicularly to the SrO 2 plane. Such elementary diffusion steps give rise to a multitude of possible pathways, the two limiting cases being the circular ( Supplementary Movie M3 ) and zig-zag ( Supplementary Movie M4 ) paths shown in Fig. 4d . It is interesting to note that a similar cooperative mechanism for fast ion conduction has been found in other oxide materials with tetrahedral moieties, for example, gallium-based oxides [25] , [26] and Si/Ge apatites [27] , where the common features are the presence of open 2D tetrahedral channels and the structural flexibility for local relaxation, as well as changes in cation coordination. 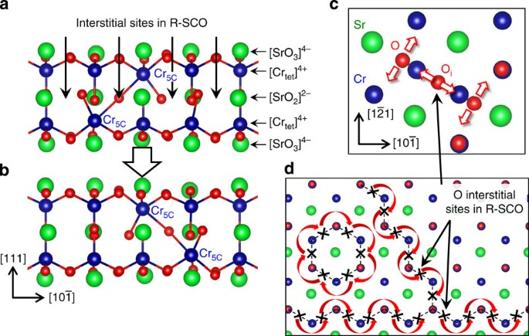Figure 4: Model of oxide anion diffusion. Geometrical configurations of an interstitial oxide ion in R-SCO before (a) and after (b) a single-diffusion event entailing the breaking of one O–Cr5Cbond and formation of another one. (c) View along the [111] direction showing a [Crtet]4+–[SrO2]2––[Crtet]4+layer in R-SCO. Four possible directions for elementary diffusion steps given by two displacement directions of interstitial oxygen (Oi) and two directions for each of the neighbouring lattice oxygen molecules. (d) Examples of oxygen diffusion pathways in the SrO2plane of R-SCO: circular and zig-zag paths. Large (green), medium (blue) and small (red) correspond to Sr, Cr and O atoms, respectively. Interstitial oxygen sites in the SrO2plane are shown with arrows inaand with crosses ind. The axis orientation inb(c) is the same as that ina(d). All Miller indices are referenced to the cubic perovskite structure of P-SCO. Figure 4: Model of oxide anion diffusion. Geometrical configurations of an interstitial oxide ion in R-SCO before ( a ) and after ( b ) a single-diffusion event entailing the breaking of one O–Cr 5C bond and formation of another one. ( c ) View along the [111] direction showing a [Cr tet ] 4+ –[SrO 2 ] 2– –[Cr tet ] 4+ layer in R-SCO. Four possible directions for elementary diffusion steps given by two displacement directions of interstitial oxygen (O i ) and two directions for each of the neighbouring lattice oxygen molecules. ( d ) Examples of oxygen diffusion pathways in the SrO 2 plane of R-SCO: circular and zig-zag paths. Large (green), medium (blue) and small (red) correspond to Sr, Cr and O atoms, respectively. Interstitial oxygen sites in the SrO 2 plane are shown with arrows in a and with crosses in d . The axis orientation in b ( c ) is the same as that in a ( d ). All Miller indices are referenced to the cubic perovskite structure of P-SCO. Full size image On the basis of these results, we propose the following model for oxygen uptake in R-SCO. Oxygen transport along the oxygen-deficient planes requires overcoming the ~0.15 eV barrier at the initial stages of R-SCO oxidation. As oxidation progresses and SrO 2 planes convert into SrO 2.25 planes, the rhombohedral structure is preserved but the lattice parameters decrease gradually. This change results in a lower diffusion barrier (0.12 eV) and, potentially, faster oxygen transport, provided that oxygen dissociation/formation of O 2− is not the rate-determining step. Once the amount of absorbed oxygen is sufficient to induce the R-to-P transition, the O 2− diffusion mechanism changes to that of an isolated V O in the perovskite bulk, and the diffusion barrier abruptly increases to 0.5 eV. Reduction back to the R phase requires a higher temperature because the fast-conducting SrO 2 planes are no longer present and some form of hopping diffusion must occur to generate sufficiently high concentration of V O , which in turn aggregate to form new SrO 2 planes. In summary, we have shown that during epitaxial growth of strontium chromite on (001)-oriented perovskite substrates, SrCrO 2.8 spontaneously nucleates to form {111}-oriented planes, and these planes exhibit fast O 2− diffusion during a reversible phase transition to SrCrO 3- δ . This structure, a 15 R polytype, is fundamentally different from those of epitaxial SrFeO 3- δ and SrCoO 3- δ , in which V O spontaneously order into alternating layers of stoichiometric octahedral and oxygen-deficient tetrahedral planes along the [001] direction, giving rise to an orthorhombic brownmillerite structure at δ =0.5 (refs 28 , 29 ). Ab initio modelling sheds considerable light on the process in which {111}-oriented domains constitute low-energy diffusion pathways that facilitate rapid oxidation of the structure, giving rise to a semiconductor-to-metal transition at low temperature. Sample preparation Epitaxial SrCrO 3- δ films with thicknesses of ~50 nm were grown by molecular beam epitaxy on two substrates: (001)-oriented LAO ( a LAO =3.796 Å) and LSAT ( a LSAT =3.868 Å). Since bulk SrCrO 3 adopts a cubic perovskite structure with a lattice constant of a p =3.819 Å (ref. 13 ), LAO substrates will impose a compressive strain of ε =−0.7%, whereas LSAT induces a tensile strain of ε =1.28% if the films remain fully coherently strained. The substrates were cleaned by annealing at 750 °C for 20 min in an oxygen partial pressure of 6 × 10 −6 Torr before film growth. Sr and Cr were evaporated from high-temperature effusion cells and the evaporation rates were calibrated using a quartz crystal microbalance positioned at the substrate position. The substrate temperature was set to 750 °C and oxygen partial pressure was kept at ~3.5 × 10 −6 Torr during growth. Reflection high-energy electron diffraction intensity oscillations and patterns were used to monitor the overall growth rate and surface structure, respectively. After film growth, the oxygen valve was closed, the gas was rapidly pumped out and the substrate temperature was lowered at a rate of 50 °C min −1 . Characterization In situ high-resolution X-ray photoemission spectra excited using monochromatic Al K α X-rays ( hν= 1,486.6 eV) were measured in a VG/Scienta SES 3000 electron energy analyser and used to determine composition, cation valence and electronic properties. The total energy resolution was 0.5 eV. The binding energy scale was calibrated using a polycrystalline Au foil in direct electrical contact with the samples. Film structures were determined using high-resolution XRD with a Philips X’Pert diffractometer equipped with a Cu anode. A hybrid monochromator, consisting of four-bounce double-crystal Ge (220) and a Cu X-ray mirror, was placed in the incident beam path to generate monochromatic Cu K α 1 X-rays ( λ =1.54056 Å) with a beam divergence of 12 arc seconds. Cross-sections of ~30–60 nm thickness were prepared with an FEI Helios dual-beam focused ion beam/scanning electron microscope using a standard lift-out approach and examined with a probe-corrected FEI Titan 80–300 TEM with a Gatan QuantumER imaging filter with dual-EELS capability, operated at 300 kV (imaging) or 80 kV (EELS), with an energy resolution of ~0.8 eV. In situ oxidation experiments were performed with an image-corrected FEI Titan 80–30 ETEM operated at 300 kV, at pressures <2 mbar and temperatures <500 °C, using a Gatan dual-tilt heating holder. Reported pressures are based upon a weighted average of Barocel and Pirani gauge readings (typical for ETEMs). Film resistivity measurements were performed using a Van der Pauw method in the temperature range of 100–300 K. Optical absorption measurements were performed at room temperature using a Cary 5000 spectrophotometer in the photon energy range of 0.4–4.5 eV. Ab initio calculations The SrCrO 3 lattice was represented using a periodic model approach. Most of the calculations were performed using a supercell with lattice vectors a 1 =2 a ( i – k ), a 2 = a ( i –2 j + k ) and a 3 =2 a ( i + j + k ), where a is the lattice parameter for cubic SrCrO 3 , and i , j and k are parallel to the [100], [010] and [001] crystallographic axes, respectively. The simulations were performed using density functional theory, the exchange-correlation functional by Perdew et al . (PBE) [30] and projector-augmented wave potentials [31] in the spin-polarized mode, as implemented in the Vienna Ab-initio Simulation Package (VASP) code [32] , [33] . The plane-wave basis with a 500-eV cutoff and a 2 × 2 × 2 Monkhorst-Pack grid were used. The supercell parameters and internal coordinates were optimized for the ideal lattice as well as for the supercell containing one, two, three and four neutral oxygen vacancies in one of the Sr 4 O 12 planes. The vacancy formation energy was calculated with respect to half the energy of a gas-phase oxygen molecule. The interaction between two isolated oxygen-deficient planes was simulated using the supercell with lattice vectors a 1 = a ( i – k ), a 2 = a ( j – k ) and a 3 =5 a ( i + j + k ). The diffusion barriers were calculated using the nudged elastic band method and eight intermediate image configurations. How to cite this article : Zhang, K. H. L. et al . Reversible nano-structuring of SrCrO 3 -δ through oxidation and reduction at low temperature. Nat. Commun. 5:4669 doi: 10.1038/ncomms5669 (2014).